Involvement of mitochondrial dynamics in the segregation of mitochondrial matrix proteins during stationary phase mitophagy Mitophagy, the autophagic degradation of mitochondria, is an important housekeeping function in eukaryotic cells, and defects in mitophagy correlate with ageing phenomena and with several neurodegenerative disorders. A central mechanistic question regarding mitophagy is whether mitochondria are consumed en masse , or whether an active process segregates defective molecules from functional ones within the mitochondrial network, thus allowing a more efficient culling mechanism. Here we combine a proteomic study with a molecular genetics and cell biology approach to determine whether such a segregation process occurs in yeast mitochondria. We find that different mitochondrial matrix proteins undergo mitophagic degradation at distinctly different rates, supporting the active segregation hypothesis. These differential degradation rates depend on mitochondrial dynamics, suggesting a mechanism coupling weak physical segregation with mitochondrial dynamics to achieve a distillation-like effect. In agreement, the rates of mitophagic degradation strongly correlate with the degree of physical segregation of specific matrix proteins. The autophagic clearance of defective or superfluous mitochondria, or mitophagy, is an important housekeeping function in eukaryotic cells [1] . In mammals, defects in mitophagy are associated with pathologies such as Parkinson’s disease, Alzheimer’s disease and type II diabetes. In yeast, a number of protocols have been developed under which mitophagy can be assayed. Mitophagy has been observed on transfer of lactate-grown (respiring) cells in nitrogen replete medium to a nitrogen starvation medium containing glucose as carbon source (which shuts down respiration in Sachharomyces cerevisiae ) [2] and on administration of rapamycin to respiring cells [3] . Mitochondrial lesions have also been reported to induce mitophagy in yeast [4] , [5] . We developed a distinct assay, stationary phase mitophagy, in which yeast cells undergo massive mitophagy in the absence of external intervention [6] . Stationary phase mitophagy shows distinct hallmarks of being a genuine quality control event and is distinct from starvation responses [7] . Using this protocol, Kanki et al . [8] , [9] and Okamoto et al . [10] carried out screens, which identified factors involved in mitophagy. Notably, these studies identified Atg32, an integral protein of the outer mitochondrial membrane that interacts with the autophagic machinery and is essential for mitophagy under all conditions. Mitochondria are widely acknowledged to be highly dynamic structures, which constantly undergo fission and fusion, effectively forming a continuous, dynamic network that is constantly changing shape and distribution. Factors required for mitochondrial fusion as well as for mitochondrial fission have been identified in yeast, and corresponding orthologues occur in animal cells [11] , [12] . In cultured mammalian cells, 85% of mitochondrial fission events result in the formation of one depolarized daughter mitochondrion and one hyperpolarized daughter mitochondrion [13] . The depolarized daughter is then given a ‘grace period’ to regain membrane potential. Mitochondria that fail to recover do not re-fuse and are autophagocytosed [13] . Pink1, a protein kinase that contains a mitochondrial-targeting sequence, and Parkin, a ring-in between ring-type E3 ubiquitin ligase, are frequently mutated in familial Parkinson’s disease [14] , [15] . Pink1 is constitutively imported into active mitochondria and degraded in the intermembrane space, in a process that depends on the presenilin-associated rhomboid-like protease (PARL) protease [16] . On loss of the mitochondrial membrane potential, Pink1 is stabilized on the outer mitochondrial membrane [17] and recruits Parkin to the mitochondrial membrane [17] , leading to the ubiquitination of select substrates, including mitofusins [18] , [19] . These results independently suggested a role of mitochondrial dynamics in the regulation of mitophagy in mammalian cells, and this was further corroborated by other groups [20] . In yeast, however, there have been conflicting reports on the role of mitochondrial dynamics in mitophagy [9] , [3] . Proteomic analyses have been used to elucidate protein dynamics during general autophagic responses [21] . We were interested in applying this approach to stationary phase mitophagy, with the aim of testing specific hypotheses regarding the possible role of mitochondrial dynamics in mediating intramitochondrial segregation mechanisms. We indeed find that different mitochondrial matrix proteins have different proclivities to undergo mitophagic degradation, implying some sort of segregation mechanism. Strikingly, these different rates clearly correlate with a physical segregation of the same proteins within the matrix, a segregation that varies with individual protein species and is at least partly dependent on mitochondrial dynamics. Mitochondrial dynamics affect the kinetics of mitophagy The role of mitochondrial dynamics in yeast mitophagy has been controversial [3] , [22] . Dnm1 is a dynamin-like protein required for mitochondrial fission [23] , [24] . Kanki et al . [9] reported loss of mitophagic activity in dnm1Δ mutants, whereas Mendl et al . [3] claimed that mitochondrial fission is dispensable for mitophagy. However, those studies used different stimuli to induce mitophagy: Kanki et al . [9] used a nitrogen starvation protocol coupled with a carbon source switch, whereas Mendl et al . [3] induced mitophagy with rapamycin, a TOR inhibitor that has far-ranging metabolic effects. We determined the effect of DNM1 deletion on stationary phase mitophagy, using ectopically expressed Idp1-green fluorescent protein (GFP) as a reporter [7] . Using fluorescence microscopy, we observe a clear defect in the vacuolar accumulation of GFP fluorescence in dnm1Δ cells ( Fig. 1a ). To quantify this effect, western blotting with anti-GFP antibody coupled with densitometry was used to compare the levels of mitophagy in the two genotypes [25] , as judged by the percentage of signal converted into free GFP on day 4 of the experiment. As shown in Fig. 1b,c , dnm1Δ cells show distinctly slower mitophagy kinetics relative to wild type (WT), with no mitophagy observed at day 3 of the incubation, and the percent of the signal that was converted into free GFP at the 4-day time point was approximately fivefold lower in the dnm1Δ mutant relative to WT ( Fig. 1c ; P <0.005, analysis of variance). This result is consistent with the data of Kanki et al . [9] A similar effect was observed in fis1Δ cells ( Supplementary Fig. S1 ), supporting the idea that mitochondrial dynamics is required for efficient mitophagy. 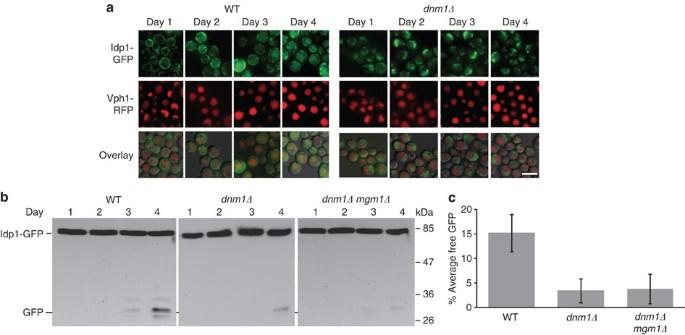Figure 1: The kinetics of stationary phase mitophagy are determined by mitochondrial dynamics, not size. (a) WT anddnm1Δcells expressing Vph1-RFP and Idp1-GFP were grown in minimal synthetic dextrose medium and transferred to lactate medium at an initial density of OD6000.08. The cells were then sampled daily and analysed by fluorescence microscopy (× 100 objective) during stationary phase mitophagy in lactate medium. Scale bar, 5 μm. (b) WT,dnm1Δanddnm1Δ mgm1Δmutants were grown in SL medium as described in Methods, and samples (10 OD600units) were taken at each time point. Protein extracts were prepared and equal protein amounts (20 μg) were subjected to SDS–polyacrylamide gel electrophoresis and immunoblotting with anti-GFP antibody. (c) Quantification of the percent free GFP at the day 4 time point in each of the three strains analysed inb, using four independent experiments for each strain. Error bars indicate s.d. analysis of variance,P<0.001;N=4. Figure 1: The kinetics of stationary phase mitophagy are determined by mitochondrial dynamics, not size. ( a ) WT and dnm1Δ cells expressing Vph1-RFP and Idp1-GFP were grown in minimal synthetic dextrose medium and transferred to lactate medium at an initial density of OD 600 0.08. The cells were then sampled daily and analysed by fluorescence microscopy (× 100 objective) during stationary phase mitophagy in lactate medium. Scale bar, 5 μm. ( b ) WT, dnm1Δ and dnm1Δ mgm1Δ mutants were grown in SL medium as described in Methods, and samples (10 OD 600 units) were taken at each time point. Protein extracts were prepared and equal protein amounts (20 μg) were subjected to SDS–polyacrylamide gel electrophoresis and immunoblotting with anti-GFP antibody. ( c ) Quantification of the percent free GFP at the day 4 time point in each of the three strains analysed in b , using four independent experiments for each strain. Error bars indicate s.d. analysis of variance, P <0.001; N =4. Full size image The observation of a significantly slower mitophagy in dnm1Δ mutants defective in mitochondrial fission may indicate that the autophagic machinery is unable to process large mitochondrial compartments [26] , or that mitochondrial dynamics functions to segregate defective components. To distinguish between these possibilities, we tested a dnm1Δ mgm1Δ double mutant. Mgm1 is a dynamin homologue that is required for mitochondrial fusion, and the double mutants have normal mitochondrial morphology but lack mitochondrial dynamics [27] , [28] , [29] . If mitochondrial size was determining the kinetics of mitophagy, then the double mutants would be expected to display increased mitophagy relative to dnm1Δ cells. Conversely, if mitochondrial dynamics is responsible, then we expect the double mutants to display kinetics similar to the dnm1Δ single mutant or even a reduced rate of mitophagy. The result, as shown in Fig. 1b,c , is consistent with mitochondrial dynamics, not mitochondrial size, as the main determinant of the rate of mitophagy under our working conditions. Proteomic analyses of protein dynamics during mitophagy We were interested in determining whether a global analysis of protein dynamics during stationary phase mitophagy could identify candidate mitochondrial proteins, which showed divergent rates of mitophagy and in testing the relationship of this discrimination to mitochondrial dynamics. To obtain a global view of stationary phase mitophagy, we adapted the stable isotope labeling with amino acids in cell culture (SILAC) protocol to yeast cells undergoing stationary phase mitophagy (see Methods and Fig. 2a ), comparing WT cells with three mutants, which are defective in different aspects of mitophagy: pep4Δ , atg32Δ, and aup1Δ ( Fig. 2b ). Pep4 is a vacuolar protease that is required for activation of zymogens in the vacuolar lumen [30] . Atg32 is an integral protein of the mitochondrial outer membrane, which is essential for mitophagy but not for other aspects of cell function, including other types of autophagy [10] , [31] . Aup1 is a mitochondrial PP2C-type protein phosphatase that is conserved between yeast and mammalian cells, and was implicated in specific aspects of stationary phase mitophagy [6] , [32] . We performed minimally two biological replicates for all experiments, and the respective quantitative proteomics data correlated well, with an overall Pearson correlation coefficient of 0.71 ( Fig. 2c , Supplementary Table S1 , Supplementary Data 1 and Supplementary Fig. S2 ). We were able to obtain good quantitative coverage with 1,551 proteins quantified in all time points in at least one yeast strain and 785 proteins with a full time course profile across all yeast strains ( Fig. 2d , Supplementary Table S1 ). 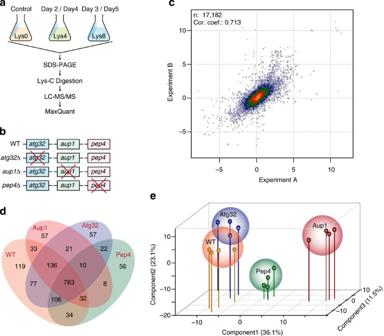Figure 2: Characterization of stationary phase mitophagy in WT and KO strains by quantitative proteomics. (a) Global protein abundance dynamics was analysed in four different ofS. cerevisiaestrains (WT,pep4Δ,atg32Δandaup1Δ) using SILAC. Global protein levels were analysed over 5-day incubations in lactate-based minimal medium. (b) To quantify changes in protein dynamics, each of the strains was labelled in lactate-based minimal media containing either normal lysine (Lys0), lysine-D4 (Lys4) or lysine-13C615N2(Lys8). Samples (10 OD600units) were taken at day 1 (Lys0), day 2 (Lys4), day 3 (Lys8), day 4 (Lys4) and day 5 (Lys8; see Methods). The mixed lysates were then separated by one-dimensional SDS–polyacrylamide gel electrophoresis and the proteins were digested with LysC. The resulting peptides were analysed by liquid chromatography-tandem mass spectrometry and the raw data were processed by MaxQuant. We performed two biological replicates of the complete time course experiments for each mutant, and three replicates for the WT, and observed good reproducibility for all the individual experiments (Supplementary Fig. S2). (c) Density plot of the reproducibility of biological replicates. (d) Venn diagram of the number of proteins identified from the different yeast strains. (e) Principal component analysis of the log2-transformed abundance changes of proteins were identified in all strains and all time points. Figure 2: Characterization of stationary phase mitophagy in WT and KO strains by quantitative proteomics. ( a ) Global protein abundance dynamics was analysed in four different of S. cerevisiae strains (WT, pep4Δ , atg32Δ and aup1Δ ) using SILAC. Global protein levels were analysed over 5-day incubations in lactate-based minimal medium. ( b ) To quantify changes in protein dynamics, each of the strains was labelled in lactate-based minimal media containing either normal lysine (Lys0), lysine-D4 (Lys4) or lysine- 13 C 6 15 N 2 (Lys8). Samples (10 OD 600 units) were taken at day 1 (Lys0), day 2 (Lys4), day 3 (Lys8), day 4 (Lys4) and day 5 (Lys8; see Methods). The mixed lysates were then separated by one-dimensional SDS–polyacrylamide gel electrophoresis and the proteins were digested with LysC. The resulting peptides were analysed by liquid chromatography-tandem mass spectrometry and the raw data were processed by MaxQuant. We performed two biological replicates of the complete time course experiments for each mutant, and three replicates for the WT, and observed good reproducibility for all the individual experiments ( Supplementary Fig. S2 ). ( c ) Density plot of the reproducibility of biological replicates. ( d ) Venn diagram of the number of proteins identified from the different yeast strains. ( e ) Principal component analysis of the log2-transformed abundance changes of proteins were identified in all strains and all time points. Full size image From Fig. 2e , it is apparent that the individual time points for each strain cluster closely together, indicating that the response of the proteome is robust across the time course for the majority of proteins. In contrast, the data from the different mutants diverge in the three dimensions of the PCA, illustrating that the mutations have distinct effects on the yeast proteome. Another observation is that atg32Δ is in close proximity to WT, whereas pep4Δ and particularly aup1Δ are more distant from the WT. This is consistent with the nature of the atg32Δ mutation, which only affects the process of mitophagic engulfment, whereas Pep4 and Aup1 have functions not restricted to mitophagy. Spatial and temporal analysis of protein level dynamics To summarize the regulation of the proteome in the four yeast strains, we subjected the pooled results to hierarchical clustering and grouped proteins with similar dynamics by k-means clustering ( Fig. 3a and Supplementary Fig. S3 ). Hierarchical clustering confirms that the atg32Δ strain is most similar to WT followed by pep4Δ , whereas aup1Δ shows the highest divergence relative to WT. The k-means clustering allowed partitioning of the proteins into five groups, each with characteristic dynamics. We tested for enrichment of gene ontology (GO) terms in each of these clusters compared with the proteins in the remaining four clusters. Distinct functional groups of proteins are enriched in each cluster ( Fig. 3a ; for graphic depiction of the clusters see Supplementary Fig. S3 ). Deletion of PEP4 and AUP1 causes an accumulation of a large group of proteins that are found in clusters 3, 4 and 5. The function of the proteins in these clusters includes mitochondrial processes but also additional cellular processes taking place in both the cytoplasm and the nucleus. In clusters 1 and 2, which contain proteins with the lowest abundance in the aup1Δ or the pep4Δ strains, we found a clear enrichment of mitochondrial proteins and processes related to mitochondrial sub-compartments. To further explore the regulation of different mitochondrial sub-compartments, we tested for significant differences in the average ratio of proteins associated with specific mitochondrial sub-compartments compared with the remaining proteins ( Fig. 3b ). We found a significant accumulation of mitochondrial matrix proteins on day 2 in the WT strain and, interestingly, this accumulation was dramatically expanded in the atg32Δ mutant. Prolonged accumulation of mitochondrial matrix proteins was also observed in the pep4Δ strain. In contrast, we observed a significant depletion of the mitochondrial intermembrane space proteins in the aup1Δ strain and no accumulation of matrix proteins on day 2. For comparison, we applied this type of analysis to proteins of the Golgi apparatus, endoplasmic reticulum (ER) and the vacuole but found no significant effect. Thus, it seems that the observed accumulation or depletion of proteins in the mitochondrial sub-compartments is specific, and is not a cell-wide phenomenon. 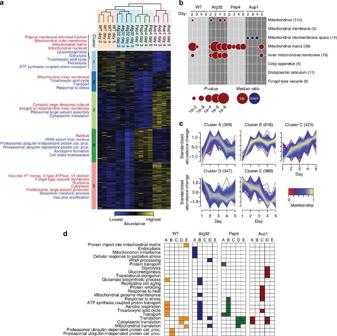Figure 3: Temporal dynamics of the yeast proteome during stationary phase mitophagy. (a) Ratios from proteins with quantifications from all samples were log2 transformed andz-score normalized. Columns containing data from the different samples were clustered hierarchically and rows that contained protein entries were clustered by k-means. The proteins in each k-means cluster were tested for enrichment of GO CC (indicated in red) and GO BP (indicated in blue) terms. (b) Proteins associated with different cellular compartments were sequentially extracted and the average of their ratios were compared with averages of remaining proteins. (c) The temporal dynamics of the protein ratios in each mutant was clustered by Fuzzy c-means. (d) GO BP enrichment analysis of proteins in the different clusters compared with the remaining proteins. Figure 3: Temporal dynamics of the yeast proteome during stationary phase mitophagy. ( a ) Ratios from proteins with quantifications from all samples were log2 transformed and z -score normalized. Columns containing data from the different samples were clustered hierarchically and rows that contained protein entries were clustered by k-means. The proteins in each k-means cluster were tested for enrichment of GO CC (indicated in red) and GO BP (indicated in blue) terms. ( b ) Proteins associated with different cellular compartments were sequentially extracted and the average of their ratios were compared with averages of remaining proteins. ( c ) The temporal dynamics of the protein ratios in each mutant was clustered by Fuzzy c-means. ( d ) GO BP enrichment analysis of proteins in the different clusters compared with the remaining proteins. Full size image To obtain a more detailed view, we clustered all time course profiles independently ( Fig. 3c ) and obtained clusters corresponding to distinct temporal dynamics. We again applied GO term enrichment analysis to assess whether particular biological processes were associated with the dynamics summarized in the clusters ( Fig. 3d ). We identified 24 GO terms that were significantly enriched. Although some were exclusive to a specific mutant, such as the upregulation of gluconeogenesis-related proteins in the aup1Δ strain, enrichment of GO terms for mitochondrial processes in clusters that were distinct from the WT profile were found in all three mutants. What particularly attracted our attention was that key mitochondrial processes such as trichloroacetic acid (TCA) cycle were enriched in different clusters (cluster B/C) in the mutants compared with the WT (cluster A). Proteins in all three clusters rapidly accumulate, but proteins in cluster A return to a level closer to the starting point on day 4, whereas proteins in clusters B/C remain at elevated levels or increase further, possibly reflecting defective mitophagy in the mutant strains. Selective mitophagic degradation and mitochondrial dynamics Proteomic analysis allowed us to identify proteins whose steady-state levels and dynamics were different between WT cells and the three mutant backgrounds. However, we cannot conclude from the SILAC data alone that these are all because of differential rates of mitophagic degradation. We chose several candidate mitochondrial matrix proteins whose levels showed extreme behaviour under these conditions, for further study. Pet9, Idh2, Idp1 and Aco2 show a decrease in abundance (when analysed in the WT background) that is not observed, or is weaker, in atg32Δ , aup1Δ and/or pep4Δ mutants. It was convenient that this group included Idp1, which we previously used the carboxy-terminally tagged version of this protein as a mitophagy marker in a plasmid-based ectopic expression system ( Fig. 1 ; ref. 7 ). In contrast, the levels of Hsp78 increase in all of the genetic backgrounds tested ( Fig. 4 ). We tagged the reading frames of these proteins with a C-terminal GFP module using the chromosomal cassette integration method [33] , utilizing transcription from the endogenous promoter to drive gene expression. We found Pet9-GFP to be non-functional, precluding it from further analysis. We scored the appearance of free GFP in the vacuolar lumen following a 7-day incubation protocol in lactate-based medium, as previously reported [7] , by western blotting with anti-GFP antibodies ( Fig. 5 ), as well as by fluorescence microscopy ( Fig. 6 ). The release of free GFP in the vacuolar lumen is an established assay for mitophagy, and is due to selective degradation of the endogenous mitochondrial protein moiety of the chimera in the vacuole [34] . Deletion of autophagy genes, such as ATG1 and ATG32, abolished the appearance of free vacuolar GFP in immunoblots and by fluorescence microscopy ( Fig. 5c and Supplementary Fig. S4 ), confirming the robustness of the assay across multiple protein chimeras and the dependence of our read-out on mitophagy. As shown in Fig. 5a , Aco2, Idp1 and Hsp78 all showed clear signs of mitophagy, as judged by the release of free GFP. However, Aco2-GFP- and Idp1-GFP-expressing cells reproducibly showed significantly higher levels of accumulated free GFP, relative to Hsp78-GFP after 7 days in respiratory medium (60 versus 20%). Idh2 on the other hand, showed extremely low levels of free GFP during these incubations (<5%), suggesting that this protein is being excluded from undergoing mitophagy. Although immunoblotting showed that the steady-state levels of Idh2 decreased with time, as predicted from the SILAC data, this decrease must occur by a non-autophagic process. One possible explanation for these data is that mitochondrial matrix proteins are segregated in a way that leads to differential rates of degradation through mitophagy. The fact that the lack of release of free GFP ( Fig. 5b ) is concomitant with a lack of appearance of vacuolar GFP ( Fig. 6 ) also rules out the possibility that the differences in the release of free GFP are due to differential susceptibility to cleavage or indirect effects on vacuole function, as in those cases we would observe vacuolar GFP even if free GFP is not observed by western blotting. 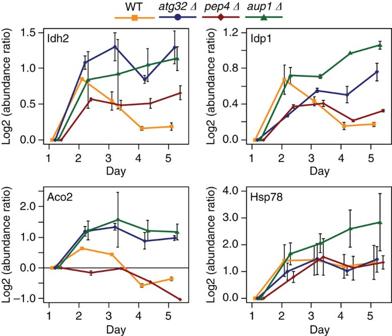Figure 4: Temporal dynamics of selected proteins. A comparison of the SILAC-derived abundance as a function of time, for several proteins that either show differential behaviour between WT and the mutants (Idh2, Idp1 and Aco2) and proteins that behave similarly between all the genetic backgrounds tested (Hsp78). Shown are mean protein ratios (two replicates for mutants, three replicates for WT), error bars indicating peptide-based relative s.d. Figure 4: Temporal dynamics of selected proteins. A comparison of the SILAC-derived abundance as a function of time, for several proteins that either show differential behaviour between WT and the mutants (Idh2, Idp1 and Aco2) and proteins that behave similarly between all the genetic backgrounds tested (Hsp78). Shown are mean protein ratios (two replicates for mutants, three replicates for WT), error bars indicating peptide-based relative s.d. 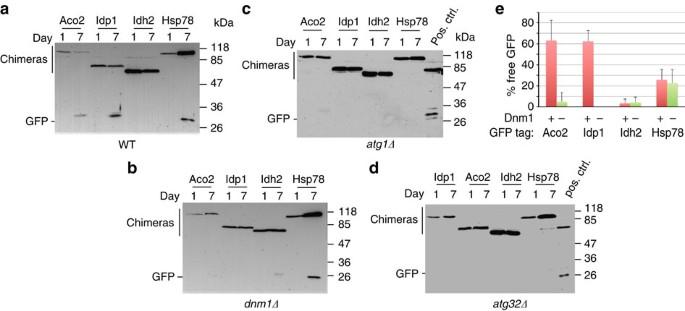Figure 5: Selective mitophagy of matrix proteins depends on mitochondrial dynamics. WT (a),dnm1Δ(b) andatg1Δcells (c) andatg32Δcells (d) expressing chromosomally tagged GFP chimeras of Aco2, Idh2, Idp1 and Hsp78 were incubated in SL medium for 7 days, and 10 OD600units were sampled at day 1 and day 7 and processed for immunoblotting with anti-GFP antibodies as described in the Methods section. Positive control used incanddwas fromdnm1Δcells expressing Idp1-GFP from a plasmid at 4-day incubation (Fig. 1b, lane 4). Release of free GFP in WT cells is reproducibly variable between these reporters, and varies between 0 (Idh2) and 60% (Aco2). (e) Densitometric quantification of the release of free GFP (as % of total signal) in four independent experiments, comparing the results between WT anddnm1Δcells. Bars denote s.d. (n=4). Full size image Figure 5: Selective mitophagy of matrix proteins depends on mitochondrial dynamics. WT ( a ), dnm1Δ ( b ) and atg1Δ cells ( c ) and atg32Δ cells ( d ) expressing chromosomally tagged GFP chimeras of Aco2, Idh2, Idp1 and Hsp78 were incubated in SL medium for 7 days, and 10 OD 600 units were sampled at day 1 and day 7 and processed for immunoblotting with anti-GFP antibodies as described in the Methods section. Positive control used in c and d was from dnm1Δ cells expressing Idp1-GFP from a plasmid at 4-day incubation ( Fig. 1b , lane 4). Release of free GFP in WT cells is reproducibly variable between these reporters, and varies between 0 (Idh2) and 60% (Aco2). ( e ) Densitometric quantification of the release of free GFP (as % of total signal) in four independent experiments, comparing the results between WT and dnm1Δ cells. Bars denote s.d. ( n =4). 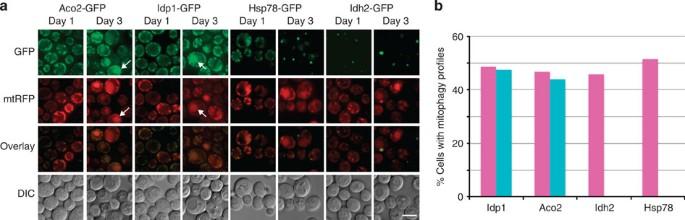Figure 6: Intramitochondrial segregation and differential mitophagic targeting. (a) Cells expressing chromosomally tagged GFP chimeras of Aco2, Idh2, Idp1 and Hsp78 as well as a plasmid-borne (pDJB12), mitochondrially targeted RFP (mtRFP) were incubated in SL-leucine medium for 3 days and imaged daily. Aco2 and Idp1 show clear mitophagic targeting (white arrows point at specific examples) by day 3, whereas Idh2 and Hsp78 show weak or no mitophagy. In addition, Idh2 and Hsp78 show different degrees of segregation relative to the mtRFP marker, whereas Idp1-GFP and Aco2-GFP show a near-complete co-localization with mtRFP. Scale bar, 5 μm. (b) Quantification of the frequency of mitophagy froma; the percentage of cells showing mitophagic profiles in the red (magenta bars; plasmid-borne mtRFP) or green (turquoise bars; integrated C-terminal GFP chimerae) was calculated for each GFP chimera. Idp-GFP, redN=76, greenN=82; Aco2-GFP, redN=79, greenN=82; Idh2-GFP, redN=72, greenN=72; Hsp78-GFP, redN=70, greenN=70. Full size image Figure 6: Intramitochondrial segregation and differential mitophagic targeting. ( a ) Cells expressing chromosomally tagged GFP chimeras of Aco2, Idh2, Idp1 and Hsp78 as well as a plasmid-borne (pDJB12), mitochondrially targeted RFP (mtRFP) were incubated in SL-leucine medium for 3 days and imaged daily. Aco2 and Idp1 show clear mitophagic targeting (white arrows point at specific examples) by day 3, whereas Idh2 and Hsp78 show weak or no mitophagy. In addition, Idh2 and Hsp78 show different degrees of segregation relative to the mtRFP marker, whereas Idp1-GFP and Aco2-GFP show a near-complete co-localization with mtRFP. Scale bar, 5 μm. ( b ) Quantification of the frequency of mitophagy from a ; the percentage of cells showing mitophagic profiles in the red (magenta bars; plasmid-borne mtRFP) or green (turquoise bars; integrated C-terminal GFP chimerae) was calculated for each GFP chimera. Idp-GFP, red N =76, green N =82; Aco2-GFP, red N =79, green N =82; Idh2-GFP, red N =72, green N =72; Hsp78-GFP, red N =70, green N =70. Full size image If mitochondrial dynamics has a role in determining the differential rates of mitophagy observed for these proteins, then the dnm1Δ mutation should produce differential effects on the GFP-tagged chimeras. As shown in Fig. 5b,e , this is indeed the case: the percentage of free GFP produced is down to 0–5% for both Aco2 and Idp1 when assayed in the dnm1Δ background, whereas it is essentially unchanged for Hsp78 (20%) and Idh2 (5%). Thus, we may conclude that mitochondrial dynamics is required for the kinetic distinction between Hsp78 and Idh2 on the one hand, and Aco2 and Idp1 on the other hand. It should also be noted that panels 5a and 5d broadly confirm the predictions of the respective proteomic analyses of WT and atg32Δ cells ( Fig. 4 ); for example, the levels of full-length Aco2-GFP clearly go down in WT but not in the mutant, whereas Hsp78 is clearly induced in all backgrounds. Physical segregation of mitochondrial matrix proteins If Hsp78 and Idh2 are kinetically distinct from Idp1 and Aco2, then, assuming our hypothesis is correct, one expects this to be reflected in some form of physical segregation. Indeed, when following the fluorescence pattern of Hsp78-GFP, Idh2-GFP, Idp1-GFP and Aco2-GFP in cells co-expressing a generic mitochondrially targeted RFP (mtRFP) from an extrachromosomal plasmid, we observe patterns that are consistent with this prediction ( Fig. 6 ). Over a 3-day incubation on synthetic lactate (SL) medium, the cytoplasmic signal of both Idp1 and Aco2, which undergoes efficient mitophagy, fully co-localizes with the mtRFP dots, indicating that they are present in an equivalent representation throughout the mitochondrial network. In addition, one observes at day 3 in these same cells the appearance of vacuolar accumulation of both RFP and GFP as predicted from the immunoblotting data. However, Idh2-GFP, which shows little or no mitophagic degradation, is distinctly restricted to one or two very brightly stained foci per cell. Although these foci co-fluoresce in red, indicating that they are part of the mitochondrial network, Idh2-GFP is clearly not evenly distributed in the network. An intriguing pattern is observed for Hsp78-GFP-expressing cells. On day 1, these cells show a uniform mitochondrial distribution that is similar to that observed for Idp1 and Aco2, with very good co-localization of the GFP and RFP signals. Gradually, however, the Hsp78-GFP signal concentrates in one or two discrete foci, which although not as powerfully bright as those observed for Idh2-GFP, represent the bulk of the cellular Hsp78 content. Again, although these foci co-fluoresce with mtRFP, the bulk of the mtRFP-positive dots do not show any significant green fluorescence by the third day of the experiment, indicating a time-dependent segregation of Hsp78 within the mitochondria, which coincides with the onset of stationary phase mitophagy. A quantification of the signal overlaps of Fig. 6a is given in Supplementary Table S1 . These results correlate with the release of free GFP in the sense that Idh2-GFP exhibits the most extreme behaviour both with regard to stability and with regard to physical segregation, while HSP78-GFP is intermediate in both cases. Idp1-GFP and Aco2-GFP, which seem to be uniformly distributed in the mitochondria, are also the most susceptible to mitophagic degradation. Interestingly, we find that the Hsp78-GFP puncta, as well as the Idh2-GFP puncta, show partial co-localization with the ER–mitochondrial-tethering complex [35] , [36] marker Mdm34 ( Supplementary Fig. S5 ). Mitochondrial dynamics affects matrix protein segregation If mitochondrial dynamics has a role in the time-dependent segregation of Hsp78-GFP, then dnm1Δ cells should show reduced segregation, as measured by the degree of co-localization of mtRFP and Hsp78. Although deletion of DNM1 does not abolish the formation of intensely fluorescent Hsp78-GFP puncta, it does quantitatively reduce the recruitment of Hsp78-GFP molecules from the general matrix milieu to these puncta, as shown by channel correlation graphs ( Fig. 7 ). In these experiments, we can see that the relative co-localization of mtRFP and Hsp78-GFP is reduced between day 1 (Pearson’s correlation coefficient 0.881) and day 3 (Pearson’s correlation coefficient 0.457). This is because of the accumulation, on day 3, of high-intensity GFP channel pixels that do not accumulate RFP fluorescence to the same extent. In contrast, dnm1Δ cells show a much milder change from a correlation coefficient of 0.85 to 0.696. Although high-intensity GFP channel pixels do accumulate in the mutant on day 3, many of them are also correlated with increased red channel fluorescence, in contrast with the situation observed in WT cells where the high-intensity regions in the green channel rarely coincide with high-intensity red regions. This result confirms that loss of the mitochondrial fission has an impact on the segregation of Hsp78-GFP from the general matrix milieu. 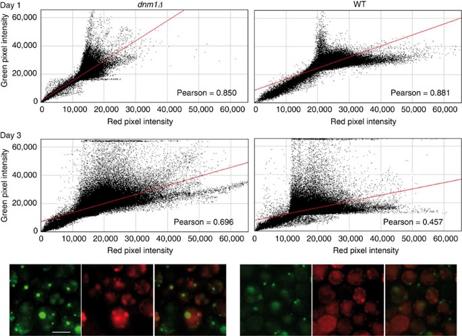Figure 7: Decreased segregation of Hsp78-GFP indnm1Δcells. WT anddnm1Δcells expressing integrated Hsp78-GFP and plasmid-borne mtRFP were grown on lactate medium for 3 days. Cells were imaged daily and the images were analysed using ImageJ as described in Methods. Graphs illustrate the distribution of pixels associated with specific values of RFP and GFP channel intensities, respectively. Diagonal concentrations of dots indicate spatial correlation between the signals. The coloured photographic panels at the bottom illustrate the increased intensity correlation of the two channels at the 3-day time point in thednm1Δmutant, relative to the WT cells. Scale bar, 5 μm. Figure 7: Decreased segregation of Hsp78-GFP in dnm1Δ cells. WT and dnm1Δ cells expressing integrated Hsp78-GFP and plasmid-borne mtRFP were grown on lactate medium for 3 days. Cells were imaged daily and the images were analysed using ImageJ as described in Methods. Graphs illustrate the distribution of pixels associated with specific values of RFP and GFP channel intensities, respectively. Diagonal concentrations of dots indicate spatial correlation between the signals. The coloured photographic panels at the bottom illustrate the increased intensity correlation of the two channels at the 3-day time point in the dnm1Δ mutant, relative to the WT cells. Scale bar, 5 μm. Full size image In this manuscript, we have identified a role for mitochondrial dynamics, as opposed to mitochondrial size, in regulating the rate of mitophagy. By comparing the dynamics of mitochondrial protein levels during stationary phase mitophagy, we found that the abundance of mitochondrial matrix proteins shows differential time-dependent behaviour during stationary phase mitophagy and that a subset of these proteins further shows differential dynamics in WT cells relative to mutants defective for different aspects of mitophagy. In the case of the proteins that were more closely analysed in this study, these differential dynamics also seem to reflect differential rates of mitophagy in WT cells ( Fig. 5 ). Thus, mitochondrial matrix proteins undergo mitophagy with differential kinetics. This result strongly supports the notion of active segregation within the matrix. How would we envisage this? One hypothesis is that mitochondrial fission and fusion are loosely coupled with a weak segregation mechanism and that on many rounds of fission and fusion, defective components will be ‘distilled’ from the network and earmarked for degradation [32] . In agreement, we find that the kinetic distinction between slowly degraded mitochondrial matrix proteins such as Idh2 and Hsp78 on the one hand, and the rapidly degraded Idp1 and Aco2 on the other hand, is clearly a function of mitochondrial dynamics ( Fig. 5 ). When using an ectopically expressed reporter, we find that the loss of mitochondrial dynamics leads to a significantly slower onset of mitophagy ( Fig. 1 ). This reduction can be uncoupled from general effects on mitochondrial morphology, as a double dnm1Δ mgm1Δ mutant does not show any signs of rescue for this phenotype ( Fig. 1c ), although it suppresses the mitochondrial morphology phenotype of the dnm1Δ mutation [27] , [28] . The segregation of Hsp78-GFP and Idh2-GFP into distinct puncta seems to partly overlap with the distribution of Mdm34, a component of the ER–mitochondrial-tethering complex [35] , [36] ( Supplementary Fig. S5 ). As the ER–mitochondria junctions have been suggested to have a role in mitochondrial fission [37] , [38] , our results may also hint at a role of these junctions in the segregation of matrix proteins. Intramitochondrial segregation of matrix proteins has been observed before, for example, with specific mutant alleles of Ilv5, a protein required both in branched amino-acid synthesis as well as in mitochondrial genome maintenance [39] . Interestingly, under some conditions the same mutant protein underwent specific, Pim1-dependent degradation that was in turn affected by Hsp78 function [39] . Hsp78 (and perhaps Idh2) segregation may also indicate localization of select proteins to sites of Pim1-dependent proteolysis. This would explain the mitophagy-independent reduction that we observe in Idh2 levels if segregation is related to Pim1-dependent degradation of Idh2. In addition, oxidized yeast aconitase segregates away from non-oxidized aconitase during mitosis, with the oxidized molecules preferentially being sequestered in the mother cell and away from the budding daughter cell [40] . One important corollary of the present study is that the outcome of any mitophagy experiment strongly depends on the nature of the reporter(s) that are chosen to represent mitophagic degradation. Even more surprising, however, is the fact that for a given individual protein, an endogenously expressed reporter can behave somewhat differently from ectopically overexpressed molecule. Note that the effect of the dnm1Δ mutation on the endogenous Idp1-GFP seems to be absolute, in the sense that no free GFP is observed even after 7 days of incubation ( Fig. 5 ). In contrast, an ectopic, overexpressed copy of Idp1 is slowly transported to the vacuole even in dnm1Δ cells ( Fig. 1 ), and free GFP is observed after 4 days. This apparent discrepancy may actually hint at an underlying segregation mechanism: if functioning mitochondrial matrix proteins are tightly ensconced in a gel-like matrix of interacting proteins, and if we assume that malfunctioning proteins are not associated with this matrix, then this distinction may provide a mechanism for a fission-coupled segregation effect. Similarly, overexpressing a protein beyond the stoichiometric balance dictated by the matrix, as we have done with Idp1-GFP in Fig. 1 , would also lead to increased accumulation of ‘unattached’ protein that would be more susceptible to mitophagic degradation even in the absence of a fully functional segregation mechanism. Although this manuscript was under revision, Mao et al . [41] published that Dnm1 directly interacts with Atg11, a component of the autophagic machinery, and that this interaction is important for efficient starvation-induced mitophagy. Although this result clearly supports a direct role for Dnm1 in regulating mitophagy, further work is required to understand how this interaction may be linked to the segregation and differential degradation of matrix components during stationary phase mitophagy. In mammalian cells, mitochondrially derived, lysosome-bound vesicles were shown to contain differential representation of mitochondrial proteins derived from different sub-compartments [42] , [43] , as well as differential representation of inner membrane electron transport chain components. Although our results also indicate a form of segregation, they are also distinct in that we find evidence for segregation of matrix proteins among themselves during mitophagy as a mechanism for selectivity. In addition, we find clear evidence for an autophagic mechanism of transport of these components to the vacuole, whereas the mechanism identified by the studies performed by Soubannier et al . [43] is clearly independent of autophagy as well as of the mammalian Dnm1 orthologue, Drp1 (refs 43 , 44 ). The recent study by Vincow et al . [45] (a comparison of that study with our results is available in Supplementary Fig. S6 ), also found variations in the degree to which different mitochondrial proteins accumulate in response to a block of mitophagy. Although that study did not demonstrate differential mitophagy of those proteins, it stands to reason that selectivity is a conserved feature of mitophagy across the eukaryotes. In support of this, a recent proteomic study of protein turnover in mouse mitochondria [46] found that the half-life of mitochondrial proteins varied from hours to months. As, in the absence of segregation, the rate of mitophagy would predict a uniform turnover in the range of hours and days [13] , one is tempted to invoke segregation and selective mitophagy in this case as well. Although it remains to be seen whether mitochondrial dynamics orchestrate a similar segregation during mammalian mitophagy, the conservation of the fission–fusion machinery, coupled with the data of Twig et al . [13] strongly suggest that these phenomena are conserved. Oligonucleotides Oligonucleotides were purchased from Hylabs (Rehovot, Israel) and the relevant sequences appear in Supplementary Table S2 . Plasmids Plasmids pHAB102 (ref. 47 ) and pDJB11 (ref. 7 ) were previously described. Plasmid pHAB129 was generated by cloning a PacI-AscI fragment from pHAB102 into PacI-AscI-digested pFA6a-kanMX6 (ref. 33 ). To generate plasmid pDJ12, the mRFP1 open reading frame (ORF) [48] was amplified with oligonuceotides F1 and R1, containing flanking Bgl II and Xho I restriction site extensions, respectively. PYX142 (ref. 49 ) was digested with Bgl II and Xho I to discard the GFP reading frame, and the gapped plasmid was ligated into the Bgl II– Xho I-digested mRFP insert to yield pDJ12. Yeast strains Deletion mutants and epitope-tagged strains were constructed by the cassette integration method [33] , using plasmids pHAB102, pHAB152 (ref. 6 ) or pFA6a-KanMX6 (ref. 33 ) as template, unless otherwise specified. Strain HAY77 ( MAT α leu2-3,112 ura3-52 his3- Δ 200 trp1- Δ 901 lys2-801 suc2- Δ 9) [50] was used as the WT standard in these studies. All knockout (KO) strains were verified by PCR. To generate strain HAY881 ( dnm1Δ ), oligonuceotides F2 and R2 (see Supplementary Table S2 ) were used to amplify the Schizosaccharomyces pombe HIS5 gene and generate a KO cassette. The PCR product was transformed into HAY77 to generate strain HAY881. To generate strain HAY706, the Vph1 ORF was C-terminally tagged with mRFP [48] . Oligonucleotides F3 and R3 were used to amplify the mRFP ORF joined to the S. pombe HIS5 gene, generating a C-terminal-tagging cassette. The amplification product was used to transform strain HAY77. To generate strain HAY1197, strain HAY706 was transformed with a KO cassette targeting dnm1, which was amplified from plasmid pHAB152 (encoding G418 resistance) using the oligonuceotides F4 and R4. Strains HAY395 ( atg1Δ ) [47] and HAY809 ( aup1Δ ) [7] were previously described. Strain HAY1097 ( atg32Δ ) was generated from HAY77 by transforming a KO cassette encoding the S. pombe HIS5 gene into the ATG32 locus. The cassette was produced by PCR, using plasmid pHAB102 as template and the oligonucleotides F5 and R5 as primers. Strain HAY1156 ( dnm1Δ mgm1Δ ) was generated from strain HAY881 by transforming with an MGM1 KO cassette encoding the S. pombe HIS5 gene and containing flanking sequences from the MGM1 ORF. The cassette was produced by PCR, using plasmid pHAB129 (encoding G418 resistance) as template and the oligonucleotides F6 and R6 as primers. Strains HAY1161, HAY1164, HAY1165 and HAY1167 were generated by transforming strain HAY77 with PCR cassettes amplified from pHAB152. The oligonucleotides used were as follows: For HAY1161, F7 and R7; for HAY1164, F8 and R8; for HAY1165, F9 and R9; for HAY1167, F10 and R10. Strains HAY1245 ( HSP78 -GFP::G418 MDM34 -RFP:: HIS5 ) and HAY1246 were generated from strains HAY1161 and HAY1167, respectively, by transforming with a PCR product amplified from plasmid pHAB147 using the oligonuceotides F11 and R11. Growth conditions Yeast were grown in synthetic dextrose medium (0.67% yeast nitrogen base, 2% glucose, auxotrophic requirements and vitamins as required) or in SL medium (0.67% yeast nitrogen base, 2% lactate pH 6, 0.1% glucose, auxotrophic requirements and vitamins as required). All culture growth and manipulations were at 26 °C unless indicated otherwise. Chemicals and antisera Chemicals were purchased from Sigma-Aldrich (Rehovot, Israel) unless otherwise stated. Custom oligonucleotides were from Hylabs or IDT (Bet Shemesh, Israel). Anti-GFP antiserum was from Santa Cruz (Dallas, TX). Horseradish peroxidase-conjugated goat anti-rabbit antibodies were from MP Biomedicals (Santa Ana, CA). Lysine-D4 and lysine- 13 C 6 15 N 2 were purchased from Silantes GmbH (Munich, Germany). Preparation of whole-cell extracts for western blot analysis Cells (10 OD 600 units) were treated with TCA (Sigma T0699) at a final concentration of 10% and washed three times with acetone. The dry cell pellet was then resuspended in 100 μl cracking buffer (50 mM Tris pH 6.8, 3.6 M urea, 1 mM EDTA, 1% SDS) and vortexed in a Disruptor Genie (Scientific Instruments, Bohemia, NY) at maximum speed with an equal volume of acid-washed glass beads (425–600 μm diameter) for 30 min. Unlysed cells were removed by centrifugation at 13,000 g for 5 min and protein was quantified using the bicinchoninic acid protein assay (Thermo Scientific, Rockford, IL). An equal volume of 2 × SDS loading buffer (100 mM Tris pH 6.8, 20% glycerol, 2% SDS, 500 mM β-mercaptoethanol) was added to the supernatant. The samples (20 μg protein per lane) were incubated at 70 °C for 5 min before loading on gels. ImageJ software was used for band quantification. Fluorescence microscopy Typically, culture samples were placed on standard microscope slides (3 μl) and viewed using a Nikon E600 upright fluorescent microscope equipped with a × 100 Plan Fluor objective, using a fluorescein isothiocyanate fluorescent filter (for viewing GFP fluorescence) or a Cy3 filter (for viewing FM4-64). To achieve statistically significant numbers of cells per viewing field in some pictures, high cell densities were achieved by sedimenting 1 ml cells for 30 s at 500 g and resuspending the pellet in 20 μl of medium. Pictures were taken with a Photometric Coolsnap charge-coupled device camera. For quantitative analysis of co-localization, we used ImageJ software with the Just Another Co-localization Plugin [51] . Representative fields, each encompassing >200 cells, were analysed in terms of channel intensity correlation by plotting cytofluorograms and calculating the Pearson correlation coefficient and Mander’s coefficients. For quantitative estimates of mitophagic trafficking, mitophagy was scored as the appearance of mitochondrial fluorescent proteins in the vacuolar lumen (defined as green fluorescence overlapping the vacuole). SILAC labelling Yeast cultures were grown to saturation in synthetic dextrose medium, washed in sterile double-distilled water and resuspended in SL lacking lysine at a density of 0.08 OD 600 . The cell suspension was divided into three equal parts. These were each supplemented with differentially isotopically substituted lysine as follows: regular lysine, lysine +4 dalton (lysine-D 4 ) and lysine +8 dalton (lysine- 13 C 6 15 N 2 ) to a final concentration of 30 mg l −1 (~200 μM). Samples (10 OD 600 units) were withdrawn daily, TCA was added to 10% (final concentration), washed three times with cold acetone and air dried. The samples from days 1, 2 and 3 were combined in equal amounts before protein extraction, as were the samples from days 1, 4 and 5. Finally, the samples were air dried. Mass spectrometry and data processing SILAC-labelled samples were dissolved in 80 μl cracking buffer with acid wash glass beads. After 30 s sonification, 20 μl SDS loading buffer were added and the pH was adjusted with 1 M NaOH. Samples were reduced (1 mM dithiothreitol) and alkylated (5.5 mM iodoacetamide). Protein mixtures were separated by SDS–polyacrylamide gel electrophoresis using 4–12% Bis‐Tris mini gradient gels (NuPAGE, Invitrogen). The gel lanes were cut into 10 equal slices, proteins therein were in‐gel digested with LysC (Wako) and the resulting peptide mixtures were desalted on StageTips (Thermo Scientific). Desalted samples were fractionated by nanoscale HPLC on an Agilent 1200 connected online to an LTQ-Orbitrap XL (Thermo Scientific). Peptides were separated over a linear gradient from 10 to 30% acrylonitrile in 0.5% acetic acid with a flow rate of 250 nl min −1 . All full-scan acquisition was done in the Fourier transform mass spectrometry part of the mass spectrometer in the range from m / z 350 to 2,000 with an automatic gain control target value of 10 6 and at resolution 60,000 at m / z 400. MS acquisition was done in data-dependent mode to sequentially perform MS/MS on the five most intense ions in the full scan in the LTQ using the following parameters. AGC target value: 5,000. Ion selection thresholds: 1,000 counts and a maximum fill time of 100 ms. Wide-band activation was enabled with an activation q =0.25 applied for 30 ms at a normalized collision energy of 35%. Singly charged and ions with unassigned charge state were excluded from MS/MS. Dynamic exclusion was applied to reject ions from repeated MS/MS selection for 45 s. All recorded liquid chromatography-tandem mass spectrometry raw files were processed together in MaxQuant [52] with default parameters. For databases, searching parameters were mass accuracy thresholds of 0.5 (MS/MS) and 6 p.p.m. (precursor), maximum two missed cleavages, carbamidomethylation as fixed modification and deamidation, oxidation and protein N-terminal acetylation as variable modifications. Enzyme specificity was LysC. MaxQuant was used to filter the identifications for a false discovery rate below 1% for peptides, sites and proteins using forward-decoy searching. Match between runs were enabled with a retention time window of 2 min. From complete proteomics experiments, 240 samples were analysed by liquid chromatography-tandem mass spectrometry. We identified 2,603 protein groups, corresponding to approximately half of all predicted yeast ORFs, with the proteins being identified on average by nine peptides covering 28% of the protein sequence. Clustering and GO enrichments analysis To compare the response with the induction across the four strains, the protein quantitation ratios from each protein from the 16 samples were log2 transformed and standardized ( z -scored), and the proteins were partitioned into five clusters by k-means clustering. For enrichment analysis, GO biological process and cellular compartment terms were retrieved from the UniProt database using GProX [53] , and Fisher’s exact test followed by Benjamini and Hochberg P -value adjustment were used to extract terms enriched in each cluster when tested against the remaining five clusters. A P -value after adjustment below 0.05 and at least five occurrences in the cluster were required to assign a GO term enriched in a cluster. To address the temporal dynamics of the induction, the ratios for the individual time points were clustered together for all strains using the fuzzy c-means algorithm using in GProX [53] with default parameters. Subsequently, for the response in each strain, the GO term enrichment analysis were performed as described above with same parameters. Accession codes: MS raw data files and respective information can be downloaded from the Peptide Atlas Data Repository ( http://www.peptideatlas.org/PASS/PASS00341 ) using the password FV8467pe [54] . How to cite this article: Abeliovich, H. et al . Involvement of mitochondrial dynamics in the segregation of mitochondrial matrix proteins during stationary phase mitophagy. Nat. Commun. 4:2789 doi: 10.1038/ncomms3789 (2013).